Cascaded optical transparency in multimode-cavity optomechanical systems Electromagnetically induced transparency has great theoretical and experimental importance in many areas of physics, such as atomic physics, quantum optics and, more recent, cavity optomechanics. Optical delay is the most prominent feature of electromagnetically induced transparency, and in cavity optomechanics, the optical delay is limited by the mechanical dissipation rate of sideband-resolved mechanical modes. Here we demonstrate a cascaded optical transparency scheme by leveraging the parametric phonon–phonon coupling in a multimode optomechanical system, where a low damping mechanical mode in the unresolved-sideband regime is made to couple to an intermediate, high-frequency mechanical mode in the resolved-sideband regime of an optical cavity. Extended optical delay and higher transmission as well as optical advancing are demonstrated. These results provide a route to realize ultra-long optical delay, indicating a significant step towards integrated classical and quantum information storage devices. The photon is the ideal choice for long-distance communication owing to its low propagation loss, high speed and large bandwidth. In both quantum and classical domains, optical delay is a favoured feature for advanced optical networks, as it offers the ability to buffer and store optical signals [1] . One promising method to produce optical delay is through the electromagnetically induced transparency (EIT) [2] , which arises from the quantum interference between different excitation paths as demonstrated in many platforms [3] , [4] , [5] , [6] , [7] . The optical transmission and delay time are the two important parameters to describe the performance of one EIT process. For example, quantum memories have been proposed based on EIT [8] , [9] , where the optical transmission and delay directly determine the information transfer efficiency and storage time [10] , [11] . EIT has also been demonstrated with cavity optomechanical systems [6] , [7] , which has advanced into the quantum regime, and paved the way to realize integrated quantum devices [12] , [13] , [14] , [15] , [16] . In spite of great advances in the performance of optomechanical devices, it remains challenging to realize EIT with both high optical transmission and long optical delay. The resolved-sideband condition requires high mechanical frequency that inevitably leads to high mechanical dissipation rate, thus small optical delay [6] , [7] . Also due to transparency window broadening under large optomechanical cooperativity [6] , [7] , the optical transmission can only be increased with at the expense of further decreased optical delay. In this article, we propose and experimentally demonstrate a cascaded EIT effect utilizing both optomechanical coupling and parametric phonon–phonon coupling [17] , in which the optical transmission and optical delay can be improved simultaneously. An aluminium nitride (AlN) wheel structure is fabricated to support whispering gallery optical modes, a low-frequency breathing mechanical mode and a high-frequency pinch mechanical mode. The parametric phonon–phonon coupling is first characterized by EIT and electromagnetically induced absorption (EIA) in the subsystem consisting of the two mechanical modes. Then by combining the optomechanical coupling and parametric phonon–phonon coupling, a secondary narrow transparency window produced by the low-frequency breathing mechanical mode is observed on the top of the original wide transparency window produced by the high-frequency pinch mechanical mode. In this cascaded EIT scheme, the optical delay is improved by eight times with simultaneous increase in optical transmission compared with normal EIT configuration. Theoretical description As shown in Fig. 1a,b , we start with a regular optomechanical system in the resolved-sideband regime, where an optical cavity (frequency ω o , linewidth κ ) is coupled to a high-frequency mechanical mode (frequency Ω H , linewidth Γ H ) with coupling rate g om . We introduce another sideband-unresolved low-frequency mechanical mode (frequency Ω L , linewidth Γ L ), which couples to the high-frequency mechanical mode through parametric phonon–phonon coupling with coupling rate g mm . The interaction Hamiltonian of the parametric phonon–phonon coupling has a similar form as radiation pressure coupling in optomechanical systems ( Supplementary Note 1 ). In cavity optomechanical systems, the photon–phonon coupling can be strongly enhanced by a coherent optical pump leading to EIT phenomena. Analogously, the subsystem consisting of the two parametrically coupled mechanical modes should also exhibit EIT phenomena [17] . 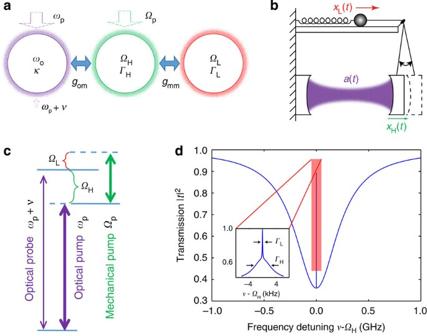Figure 1: Cascaded EIT model. (a) Schematic of the multimode coupling scheme. The optical and mechanical pumps are positioned atωpand Ωp, respectively, and a weak optical probe is located atωp+ν. (b) A model of the multimode coupling. One mirror of the Fabry–Perot cavity (the optical cavity) is suspended from a pivot, forming a pendulum (the high-frequency mechanical mode), and the length of the pendulum (hence the frequency) is determined by the position of a small ball attached to a spring (the low-frequency mechanical mode). (c) The energy-level diagram of the multimode coupling scheme. The optical pump frequency isωp=ωo−ΩH, and the mechanical pump frequency is Ωp=ΩH+ΩL. (d) Calculated transmission spectrum of the probe light (equation (3)) as a function of the probe light frequencyν. The inset reveals the ultra-narrow cascaded transparency window induced by the multimode coupling. The parameters used areωo=2π× 194 THz,κ=2π× 0.5 GHz,κex=0.2κ; ΩH=2π× 1 GHz, ΓH=2π× 20 kHz; ΩL=2π× 80 MHz, ΓL=2π× 2 kHz;gom|α0|=2π× 1.5 MHz,gmm|β0|=2π× 3 kHz. Figure 1: Cascaded EIT model. ( a ) Schematic of the multimode coupling scheme. The optical and mechanical pumps are positioned at ω p and Ω p , respectively, and a weak optical probe is located at ω p + ν . ( b ) A model of the multimode coupling. One mirror of the Fabry–Perot cavity (the optical cavity) is suspended from a pivot, forming a pendulum (the high-frequency mechanical mode), and the length of the pendulum (hence the frequency) is determined by the position of a small ball attached to a spring (the low-frequency mechanical mode). ( c ) The energy-level diagram of the multimode coupling scheme. The optical pump frequency is ω p = ω o −Ω H , and the mechanical pump frequency is Ω p =Ω H +Ω L . ( d ) Calculated transmission spectrum of the probe light (equation (3)) as a function of the probe light frequency ν . The inset reveals the ultra-narrow cascaded transparency window induced by the multimode coupling. The parameters used are ω o =2 π × 194 THz, κ =2 π × 0.5 GHz, κ ex =0.2 κ ; Ω H =2 π × 1 GHz, Γ H =2 π × 20 kHz; Ω L =2 π × 80 MHz, Γ L =2 π × 2 kHz; g om | α 0 |=2 π × 1.5 MHz, g mm | β 0 |=2 π × 3 kHz. Full size image We use the following Hamiltonian to describe the coupled multimode system: Here a , b , and c are the annihilation operators of the optical cavity, high- and low-frequency mechanical modes, respectively, and g om ( g mm ) represents the zero-point optomechanical (parametric phonon–phonon) coupling rate. In the presence of an optical pump (which results in a coherent optical field α 0 ) at the red side of the optical cavity and a mechanical pump ( β 0 ) at the blue side of the high-frequency mechanical mode, the interaction Hamiltonian is found by substituting a →( α 0 + a ), b →( β 0 + b ) under the rotating wave approximation If a weak optical probe is swept across the optical cavity, the first term in equation (2) causes destructive interference between the probe photons and the pump photons scattered by the high-frequency mechanical mode phonons, inducing transparency in the transmitted probe light [6] , [7] . The second term causes constructive interference between the high-frequency mechanical mode phonons and the mechanical pump scattered by the low-frequency mechanical mode phonons. The energy-level diagram of this cascaded EIT scheme is shown in Fig. 1c . There are three pathways for the optical probe in the cavity: (i) directly transmitting through the optical cavity, (ii) interfering with the optical pump scattered by the high-frequency mechanical mode and (iii) interfering with the optical pump scattered by the phonons scattered from the mechanical pump by the low-frequency mechanical mode. The total transmitted signal of the optical probe can be written as ( Supplementary Note 2 ) where ω p and Ω p are the optical and mechanical pump frequencies, respectively, κ ex is the optical coupling loss and ν is the frequency difference between the optical pump and probe ( Fig. 1c ). Besides the transparency window produced due to the high-frequency mechanical mode, the feature of the low-frequency mechanical mode is also imprinted in the optical probe through the parametric phonon–phonon coupling with the high-frequency mechanical mode serving as a bridge. To observe the cascaded EIT, the resolved-sideband condition is required individually for the optomechanical coupling (Ω H > κ ) and parametric phonon–phonon coupling (Ω L >Γ H ), but does not restrict the low-frequency mechanical mode to be in the resolved-sideband regime with respect to the optical cavity. Therefore, it can be designed to have lower frequency that offers a much smaller linewidth than the high-frequency mechanical mode, and leads to prolonged group delay ( Fig. 1d ). Device design and characterization The parametric phonon–phonon coupling is a key part in the cascaded EIT, which we implement in a microwheel structure ( Fig. 2a ). A displacement of one mechanical mode leads to tension and boundary change in the structure, thus modifying the resonant frequencies of other mechanical modes. Unlike the coupling induced by the Duffing effect in flexural beams where the frequency shift is proportional to the square of the displacement [18] , [19] , the frequency shift for the radial modes in microwheel structures is linearly proportional to the displacement because of the broken-mirror symmetry in the radial direction. 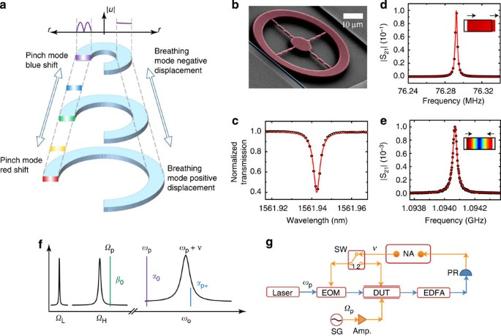Figure 2: Experimental system for studying cascaded EIT. (a) Parametric phonon–phonon coupling mechanism with pinch and breathing modes in a wheel structure. The breathing mode is depicted in the deformed shapes with three different displacements. The pinch mode is depicted as the cross-section profile (the saturation corresponds to the radial displacement amplitude). The decrease and increase of the radius cause opposite frequency changes of the pinch mode. (b) Scanning electron microscope image of the device in false colour. The inner and outer radii of the AlN wheel are 20 and 25 μm, respectively. (c) Transmission spectrum of the optical whispering gallery mode at 1,561.94 nm. (d) Driven response of the breathing mode. (e) Driven response of the pinch mode. The insets ind,eshow the displacement profiles of the wheel cross-section for each mechanical mode. (f) Configuration of the coherent signals, optical and mechanical resonances in the experiment. (g) The measurement setup. Amp, amplifier; EDFA, erbium-doped fibre amplifier; EOM, electro-optic modulator; PR, photoreceiver; SG, signal generator; SW, RF switch. The coupling rate in equations (1) and (2) can be expressed as ( Supplementary Note 1 ): Figure 2: Experimental system for studying cascaded EIT. ( a ) Parametric phonon–phonon coupling mechanism with pinch and breathing modes in a wheel structure. The breathing mode is depicted in the deformed shapes with three different displacements. The pinch mode is depicted as the cross-section profile (the saturation corresponds to the radial displacement amplitude). The decrease and increase of the radius cause opposite frequency changes of the pinch mode. ( b ) Scanning electron microscope image of the device in false colour. The inner and outer radii of the AlN wheel are 20 and 25 μm, respectively. ( c ) Transmission spectrum of the optical whispering gallery mode at 1,561.94 nm. ( d ) Driven response of the breathing mode. ( e ) Driven response of the pinch mode. The insets in d , e show the displacement profiles of the wheel cross-section for each mechanical mode. ( f ) Configuration of the coherent signals, optical and mechanical resonances in the experiment. ( g ) The measurement setup. Amp, amplifier; EDFA, erbium-doped fibre amplifier; EOM, electro-optic modulator; PR, photoreceiver; SG, signal generator; SW, RF switch. Full size image Here u H and u L are the normalized mechanical mode profiles, and are the strain tensors, C is the fourth-order elasticity tensor, ρ is the material density and u L,zpm is the zero-point motion of the low-frequency mode. The first term accounts for the potential energy change of the high-frequency mode due to the low-frequency mode displacement, and the second term accounts for the fact that the two mechanical modes are not orthogonal when structure deformation is considered. Note that the parametric phonon–phonon coupling is an intrinsic property in multimode mechanical devices, unlike the coupling induced by external electric and optical fields [20] , [21] , [22] . The efficient piezoelectric drive of mechanical resonators makes multimode-cavity piezo-optomechanical systems an ideal platform to realize our cascaded EIT [23] , [24] . We use an on-chip AlN wheel structure to obtain high- Q optical and mechanical modes, as well as high piezoelectric driving efficiency [23] , [24] ( Fig. 2b ). As an added benefit, the piezoelectric effect in AlN further enhances the parametric phonon–phonon coupling by effectively stiffening the material ( Supplementary Note 1 ). The device optimization and fabrication process are shown in Supplementary Note 3 . The optical whispering gallery mode around 1,561.94 nm wavelength has a loaded Q of 380,000, corresponding to κ =2 π × 0.51 GHz ( Fig. 2c ). The mechanical modes are characterized by piezoelectrically actuating the device and optically detecting the response in a liquid helium cryostat at temperature T =4.6 K ( Fig. 2d,e ). The two mechanical modes used in the experiment are the breathing mode (Ω L =2 π × 76.29 MHz, Γ L =2 π × 2.7 kHz) and the pinch mode (Ω H =2 π × 1.094 GHz, Γ H =2 π × 33.6 kHz), and the corresponding zero-point phonon–phonon coupling rate is 2 π × 0.028 Hz. This coupling rate can be greatly enhanced by a coherent mechanical pump that could provide a large number of phonons. The pinch mode has a frequency significantly larger than the linewidth of the optical cavity, and the same holds for the breathing mode frequency compared with the linewidth of the pinch mode, so both satisfy their respective resolved-sideband requirement. Also the breathing mode frequency is significantly small compared with the optical cavity linewidth, thus in the optomechanical unresolved-sideband regime. The optomechanical coupling between the optical mode and the low-frequency breathing mode is negligible under the rotating wave approximation due to the frequency mismatch. Parametric phonon–phonon coupling We first examine the EIT in the subsystem consisting of the two mechanical modes induced by the parametric phonon–phonon coupling. No optical pump is used, and a weak mechanical probe ( β 1 ) with frequency ν is swept across the high-frequency mechanical mode, whose motion is detected using a weak optical readout. Without phonon–phonon coupling, one simply measures the Lorentzian-driven response of the high-frequency mode as shown in Fig. 2e . With the co-existing strong mechanical pump ( β 0 ) and weak mechanical probe ( β 1 ), the radiation-like force due to the parametric phonon–phonon coupling introduces phonons into the low-frequency mechanical mode, as it drives the resonator at the frequency difference between β 0 and β 1 . These phonons in turn scatter the mechanical pump, which interfere with the mechanical probe. This EIT effect results in a sharp dip at ν =Ω H in Fig. 3a when the mechanical pump is placed at Ω p =Ω H −Ω L . The five panels in Fig. 3b show the normalized mechanical probe signal when the mechanical pump frequency is varied from Ω H −Ω L −2Γ H to Ω H −Ω L +2Γ H . The transparency window always occurs at frequency ν =Ω p +Ω L with a maximum transparency window achieved at Ω p =Ω H −Ω L . When the mechanical pump is placed at the blue side of the high-frequency mechanical mode, an absorption peak manifests itself indicating an increased phonon number in the high-frequency mechanical mode ( Fig. 3c ). 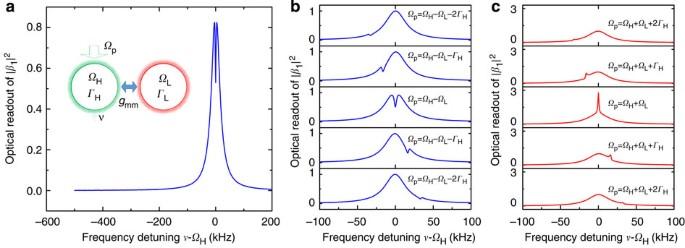Figure 3: Parametric phonon–phonon coupling in the subsystem consisting of the two mechanical modes. (a) The optically transduced high-frequency mechanical probe (|β1|2) when the mechanical pump is placed at Ωp=ΩH−ΩL. The sharp dip atv=ΩHcharacterizes the EIT phenomenon induced by parametric phonon–phonon coupling between the two mechanical modes. (b) Zoom-in of the transparency window with adjusted detuning on the red side of the high-frequency mechanical mode. (c) Zoom-in of the absorption window with mechanical pump detuned on the blue side of the high-frequency mechanical mode. Figure 3: Parametric phonon–phonon coupling in the subsystem consisting of the two mechanical modes. ( a ) The optically transduced high-frequency mechanical probe (| β 1 | 2 ) when the mechanical pump is placed at Ω p =Ω H −Ω L . The sharp dip at v =Ω H characterizes the EIT phenomenon induced by parametric phonon–phonon coupling between the two mechanical modes. ( b ) Zoom-in of the transparency window with adjusted detuning on the red side of the high-frequency mechanical mode. ( c ) Zoom-in of the absorption window with mechanical pump detuned on the blue side of the high-frequency mechanical mode. Full size image Cascaded optical transparency By combining the parametric phonon–phonon coupling and optomechanical coupling, the cascaded EIT effect can be observed. When the optical probe is swept across the optical cavity over a wide range, we first see the normal EIT that has a transparency window with a linewidth equal to the dissipation rate of the high-frequency mechanical mode ( Fig. 4a ). On zooming into the transparency window, a second transparency window sitting on top of the original transparency window can be observed ( Fig. 4b ). In this case, the linewidth of the narrow transparency window equals to the dissipation rate of the low-frequency mechanical mode instead of the much larger linewidth of the high-frequency mode. The high-frequency mechanical mode essentially mediates the coupling between the optical cavity and the low-frequency mechanical mode, which is in the optomechanical unresolved-sideband regime and therefore cannot be used for regular EIT. By fitting the spectrum in Fig. 4b with equation (3), we can obtain both the optomechanical cooperativity , and the phonon–phonon coupling cooperativity . Both cooperativities are close to unity allowing the observation of the cascaded EIT. The narrow optical transparency window leads to strong optical phase modulations as shown in Fig. 4b and therefore large optical group delays, which in our case reach 5.0 μs. This corresponds to a more than eight times improvement compared with 0.6 μs delay of the regular EIT, which only involves the high-frequency mode ( Fig. 4d ). Moreover, the optical transmission is increased, and this leads to a 10 times improvement in the bandwidth-delay product [9] . By placing the mechanical pump on the red side of the high-frequency mechanical mode, we turn the narrow peak into a dip ( Fig. 4c ). This gives rise to the advanced light with a leading time of 1.03 μs ( Fig. 4d ). 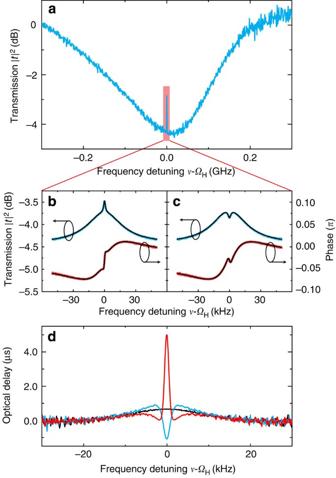Figure 4: Cascaded EIT. (a) The probe light transmission (|αp+|2) over the broad-frequency range. (b) Zoom-in of the transmission (cyan) and phase (red) of the transparency window when the mechanical pump is placed on the blue side (Ωp=ΩH+ΩL). This is the configuration for the prolonged optical delay. (c) The zooming-in transmission (cyan) and phase (red) of the transparency window when the mechanical pump is placed on the red side (Ωp=ΩH−ΩL). This is the configuration for the enhanced optical advancing. The black lines inb,care the best-fitting curves of our cascaded EIT theory. (d) The optical delay for the normal EIT configuration (black), cascaded EIT with the prolonged optical delay configuration as inb(red) and cascaded EIT with the enhanced optical advancing configuration as inc(cyan). Figure 4: Cascaded EIT. ( a ) The probe light transmission (| α p+ | 2 ) over the broad-frequency range. ( b ) Zoom-in of the transmission (cyan) and phase (red) of the transparency window when the mechanical pump is placed on the blue side (Ω p =Ω H +Ω L ). This is the configuration for the prolonged optical delay. ( c ) The zooming-in transmission (cyan) and phase (red) of the transparency window when the mechanical pump is placed on the red side (Ω p =Ω H −Ω L ). This is the configuration for the enhanced optical advancing. The black lines in b , c are the best-fitting curves of our cascaded EIT theory. ( d ) The optical delay for the normal EIT configuration (black), cascaded EIT with the prolonged optical delay configuration as in b (red) and cascaded EIT with the enhanced optical advancing configuration as in c (cyan). Full size image For optomechanical applications in information processing, one major obstacle is the short phonon lifetime that introduces noise during state transfer and limits the information storage time after state transfer [25] , [26] , [27] , [28] . In our optomechanical system, the phonon lifetime for the high-frequency mechanical mode is around 30 μ s . The phonon lifetime can be greatly increased in the cascaded multimode coupling scheme. In this scheme, the low-frequency mechanical mode in the optomechanical unresolved-sideband regime functions as if it is in the optomechanical resolved-sideband regime, and the frequency just needs to exceed the linewidth of the high-frequency mechanical mode (~33 kHz). For a mechanical resonator with frequency around 200 kHz, a linewidth as low as 0.1 Hz can be realized, corresponding to a 10-s phonon lifetime [29] . This increase in phonon lifetime is directly proportional to the information storage time increase for a classical signal. Also a higher mechanical Q can be expected for a lower-frequency mechanical mode [30] due to the empirical f · Q limit [31] . Therefore, the low-frequency mechanical mode can preserve the quantum state much longer due to its longer rethermalization time τ = ħQ / kT (ref. 32 ), thus serving as a better quantum register [33] . In essence, our cascaded coupling scheme provides a viable route to long optical delay and long coherence time by leveraging the parametric phonon–phonon coupling, pushing forward the frontier of optomechanical devices in both classical and quantum regime. Measurement setup The experiment is realized with the setup shown in Fig. 2g . In the experiment demonstrating parametric phonon–phonon coupling ( Fig. 3 ), the RF signal from a network analyzer (NA) goes through port 2 of the RF switch (SW) and is sent into the device under test (DUT) to serve as the weak mechanical probe ( β 1 ). The mechanical pump ( β 0 ) is provided by the amplified RF signal from a signal generator (SG). No optical pump is used in this part of the experiment and only a fixed weak readout laser is delivered to the DUT to linearly transduce the mechanical signal. The transmitted optical signal is amplified by an erbium-doped fibre amplifier and detected by a photoreceiver. Then the electrical signal is sent back to the NA. In the experiment demonstrating cascaded EIT ( Fig. 4 ), the optical pump ( α 0 ) from a laser is delivered to the DUT after passing through an electro-optic modulator. The RF signal from the NA goes through port 1 of the switch to modulate the strong optical pump, and this generates a weak optical probe ( α p+ ). In this case, the only RF signal sent into the device is the mechanical pump ( β 0 ), which is provided by the amplified RF signal from signal generator. The transmitted optical signal is amplified by the erbium-doped fibre amplifier and detected by the photoreceiver. Then the signal is sent back to the NA. How to cite this article: Fan, L. et al. Cascaded optical transparency in multimode-cavity optomechanical systems. Nat. Commun. 6:5850 doi: 10.1038/ncomms6850 (2015).